Sequencing trait-associated mutations to clone wheat rust-resistance geneYrNAM Stripe (yellow) rust, caused by Puccinia striiformis f. sp. tritici ( Pst ), can significantly affect wheat production. Cloning resistance genes is critical for efficient and effective breeding of stripe rust resistant wheat cultivars. One resistance gene ( Yr10 CG ) underlying the Pst resistance locus Yr10 has been cloned. However, following haplotype and linkage analyses indicate the presence of additional Pst resistance gene(s) underlying/near Yr10 locus. Here, we report the cloning of the Pst resistance gene YrNAM in this region using the method of sequencing trait-associated mutations (STAM). YrNAM encodes a non-canonical resistance protein with a NAM domain and a ZnF-BED domain. We show that both domains are required for resistance. Transgenic wheat harboring YrNAM gene driven by its endogenous promoter confers resistance to stripe rust races CYR32 and CYR33. YrNAM is an ancient gene and present in wild wheat species Aegilops longissima and Ae. sharonensis ; however, it is absent in most wheat cultivars, which indicates its breeding value. Wheat stripe (yellow) rust, caused by Puccinia striiformis f. sp. tritici ( Pst ), can be a devastating wheat disease and poses a threat to global production [1] . Cloning resistance genes in wheat is essential for studying wheat-rust interactions and can expedite wheat breeding to combat stripe rust. However, of the 86 yellow rust ( Yr ) resistance loci reported in wheat, only seven Yr genes have been cloned [2] , mostly through map-based cloning. Yr10 , derived from Turkish wheat ‘PI 178383’, was transferred to wheat cultivars ‘Moro’ [3] and AvSYr10NIL [4] , and confers all-stage resistance to Pst . Wheat cultivars with Yr10 are resistant to multiple Pst strains, including CYR29, CYR31, CYR32, and CYR33, but are susceptible to CYR34 [4] , [5] , [6] . Laroche and colleagues previously reported that a CC-NBS-LRR gene (Genbank AF149112) was a candidate for Yr10 [7] , [8] . Their conclusion is based on experimental evidence that transformation of the Pst -susceptible cultivar ‘Fielder’ with AF149112 conferred resistance to Pst race SRC-84 but not to Pst race CDL-29, which is a fairly old race and equivalent to PSTv23 (synonym, PST-29) (according to personal communications with Dr. Xianming Chen). We previously performed haplotype and linkage analyses for AF149112, which we called Yr10 CG , and found that it was 1.2 cM away from the locus conferring resistance to mixed Pst spores of CYR29, CYR31, and CYR32 [9] , [10] . Because transgenic wheat harboring AF149112 was susceptible to CYR29 [10] , a gene or locus other than Yr10 CG in the mapping region may confer resistance to CYR29. Historically, resistance genes and other genes of interest were mostly cloned using a map-based cloning strategy, which requires genetic and physical maps and is tedious and time-consuming. But fine mapping around recombination suppression regions, where most alien resistance genes localize, is difficult. In contrast to map-based cloning, DNA and/or RNA sequencing-based methods use independent mutants to clone candidate genes. These methods target specific chromosomes or specific gene classes and thus avoid the interference of the rest of the genome. In addition, these methods do not require a genetic map. Recently, several rust-resistance genes have been cloned using sequencing-based methods. For example, Yr7 , Yr5 / YrSP , Sr22 , Sr26 , Sr45 , and Sr61 were cloned by MutRenSeq [11] , [12] , [13] ; Sr43 was cloned using the MutChromSeq method [14] , [15] ; and Sr62 was cloned by MutRNA-Seq [16] . However, each of these methods has different limitations. For example, MutRenSeq is only useful for nucleotide binding and leucine-rich repeat (NLR) gene cloning; MutChromSeq has a technically-demanding step of chromosome sorting by flow cytometry; and MutRNA-Seq requires a high-quality genome assembly of the wild-type (WT). Here, we report the cloning of wheat stripe rust resistance gene YrNAM using the method of sequencing trait-associated mutations (STAM). STAM uses full-length isoform sequencing (Iso-Seq) of the WT as the reference and employs transcriptome sequencing of relevant mutants for gene cloning. We show that YrNAM encodes a protein with a NAM domain and a ZnF-BED domain. YrNAM is absent in most wheat cultivars but present in wild wheat species Aegilops longissima and Ae. sharonensis . STAM can clone genes of interest with mutants and RNA-Seq To perform STAM, full-length WT transcripts are used to generate a reference of non-redundant transcripts. Then, RNA-Seq reads of loss-of-function mutants are mapped onto the reference, variants are called, and counts of mutated transcripts are tallied (Fig. 1a ). In this study, a Pst -resistant WT P10–46 [10] and seven Pst -susceptible M 3 lines (Fig. 1b ) were used to perform STAM. Using the leaf transcriptome of the WT, we assembled 123,178 full-length non-concatemer (FLNC) isoforms, which contained our 40,564 non-redundant reference transcripts. After completing STAM, a total of 7434 mutation sites (G → A and C → T) were identified in the seven susceptible mutants. 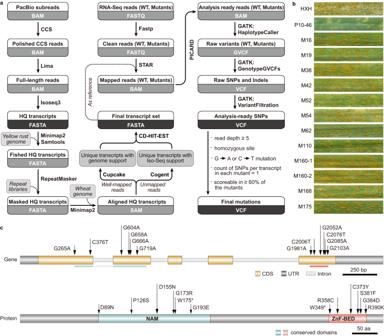Fig. 1: Identification ofYrNAMin wheat using STAM. aPipeline of STAM analysis.bResponse toPst(a mixture of races CYR29, CYR31, and CYR32) of the susceptible control cultivar ‘Huixianhong’ (HXH), the resistant wild-type P1046 withYr10, and 12Pst-susceptible mutants that were derived from EMS-treated P10–46.cGene (1737 bp) and protein structure ofYrNAM(T59230) and EMS-induced mutations in the NAM and ZnF-BED domains in the 12 mutant lines. The positions of the mutation sites are relative to ‘ATG’ or methionine. Only one transcript (T59230), was mutated in six of seven susceptible mutants (Table 1 ), i.e., all except M62. M62 segregated for Pst resistance; the Pst -susceptible segregant also has a G → A transition in T59230. Furthermore, T59230 is mutated in the other five susceptible mutants that were not submitted for RNA-Seq. Collectively, all 12 susceptible mutants have mutations in T59230 (Fig. 1c ). Thus, T59230 is the candidate for stripe rust resistance. Fig. 1: Identification of YrNAM in wheat using STAM. a Pipeline of STAM analysis. b Response to Pst (a mixture of races CYR29, CYR31, and CYR32) of the susceptible control cultivar ‘Huixianhong’ (HXH), the resistant wild-type P1046 with Yr10 , and 12 Pst -susceptible mutants that were derived from EMS-treated P10–46. c Gene (1737 bp) and protein structure of YrNAM (T59230) and EMS-induced mutations in the NAM and ZnF-BED domains in the 12 mutant lines. The positions of the mutation sites are relative to ‘ATG’ or methionine. Full size image Table 1 STAM results using Iso-Seq data from resistant WT P10–46 and RNA-Seq data from seven susceptible mutants Full size table YrNAM is a stripe rust resistance gene with NAM and ZnF-BED domains We performed DNA resequencing of P10–46 and de novo assembled ~1.1 M contigs of non-repetitive DNA with 1.8 Gb in total. Contig NODE_33935 (5633 bp, Supplementary Data 1 ) matches T59230 perfectly. T59230 CDS is 1227 bp in length and, by sequence alignment, is comprised of five exons (Fig. 1c ). The predicted protein YrNAM has a NAM (No Apical Meristem) domain ( E -value 2.7e−11) and a ZnF-BED (BED Zinc Finger) domain ( E -value 2.5e−08) at the N and C termini, respectively. The YrNAM-GFP fusion protein is expressed in nuclei in tobacco leaves (Supplementary Fig. 1 ). Mutational analysis suggests that both NAM and ZnF-BED domains are required for resistance; six of the 12 loss of function EMS mutants have a mutation in the NAM domain, and the other six have one in the ZnF-BED domain (Fig. 1c ). YrNAM co-segregates with the rust resistance in WT P10–46 To further validate that YrNAM confers stripe rust resistance in WT P10–46, we created an F 2 population using P10–46 and one Pst -susceptible mutant M19. The C2076T mutation of YrNAM in M19 was used to develop a unique diagnostic marker YrNAM-F8R2 ( Hpy188 III digestion). As expected, 113 F 2 seedlings segregated as 3:1 for stripe rust resistance and susceptibility ( χ 2 = 1.30, df = 1, P = 0.25); YrNAM-F8R2 was completely linked to stripe rust susceptibility (Supplementary Data 2 ). Previously, while re-mapping the Yr10 region, we developed a small population of 126 F 2:3 plants [10] and a fine-mapping population of 7177 F 2:5 plants [10] . Among the 126 F 2:3 plants, the dominant PCR marker YrNAM-F8R7 , which amplifies a 698 bp fragment of the 3′-end of YrNAM , completely links to the stripe rust resistance and the Yr10 co-segregating marker Xsdauw79 (Supplementary Data 3 ). Using 37 recombinants in the Xpsp3000 - Xsdauw79 interval obtained from the fine-mapping population [10] , we showed that YrNAM-F8R7 co-segregates with the stripe rust resistance derived from Moro (Supplementary Data 4 ). Transgenic YrNAM confers resistance to stripe rust We constructed a native expression vector of YrNAM (PC1213) (Fig. 2a ) and transformed it into Fielder and CB037, which are both susceptible to wheat stripe rust. Twenty T 1 seeds per line of three lines, including Fielder#3, CB037#4, and CB037#5, were tested with Pst race CYR32. The infection type (ITs) of each T 1 was correlated with the expression of YrNAM (Fig. 2b, c , Supplementary Data 5 ). The YrNAM -expressing T 1 plants in both Fielder and CB037 were immune (ITs = 0) or highly resistant (ITs = 1–2) to CYR32, while the YrNAM non-expressing T 1 and the negative control plants were highly susceptible (ITs = 7–8) (Fig. 2b, c ). YrNAM expression from genetic complementation also conferred high resistance in two additional trials (Supplementary Fig. 2 , Supplementary Data 5 ). In the T 2 generation, PC1213 transgenic plants showed resistance to CYR33, an avirulent race for YrNAM as documented in Moro, P8–13, and P10–46 (Fig. 3a ). However, CYR34 is virulent to YrNAM because it caused abundant sporulation in Moro, P8–13, and P10–46 (Fig. 3b ). Unexpectedly, PC1213 transgenic T 2 plants were resistant (ITs = 2) to CYR34 (Fig. 3b ), which may have been caused by stacking YrNAM with Yr6 in Fielder [17] and Yr9 in CB037 [18] . The WT Fielder is moderately resistant to CYR34, as indicated by a modest hypersensitive response (HR) (Fig. 3b ). Fig. 2: Genetic complementation demonstrates that YrNAM confers stripe rust resistance. a Native expression vector PC1213 was constructed for genetically transforming recipients with YrNAM . b Leaves with either a hypersensitive response (HR) or Pst -sporulation in resistant and susceptible genotypes, respectively. 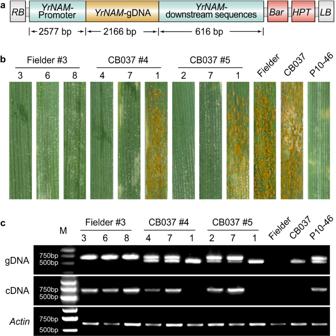Fig. 2: Genetic complementation demonstrates thatYrNAMconfers stripe rust resistance. aNative expression vector PC1213 was constructed for genetically transforming recipients withYrNAM.bLeaves with either a hypersensitive response (HR) orPst-sporulation in resistant and susceptible genotypes, respectively. Stripe rust-susceptible Fielder and CB037 were transformed withYrNAM. Nine T1plants are shown on the left. P10–46 is thePst-resistant control. Plants were inoculated withPstrace CYR32.cThe integration (genomic DNA, or gDNA) and expression (cDNA) ofYrNAM. Samples pair with those in (b). The target band for gDNA genotyping with primer pairYrNAM-F8R7is 698 bp; the smaller band (572 bp) in P10–46 and CB037 is amplified from the chromosome 1D homolog, which does not haveYrNAM.YrNAM-F4R43was used for cDNA expression with a target band of 676 bp. ThePsttest for T1plants using CYR32 was performed three times independently with similar results. Source data are provided as a Source Data file. 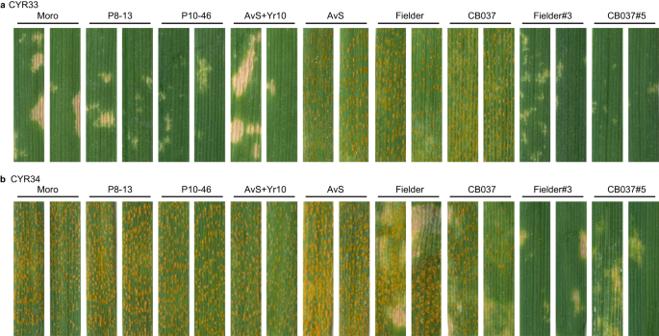Fig. 3: Reaction types ofYrNAM-containing materials to the avirulent and virulentPstraces. aYrNAM-avirulent race CYR33. Moro, P8–13, P10–46, and AvSYr10NIL (AvS +Yr10), andYrNAM-transgenic Fielder#3 and CB037#5 are resistant with obvious HR (ITs = 2), while Avocet S (AvS) and the non-transformed Fielder and CB037 are susceptible (ITs = 7–9).bYrNAM-virulent race CYR34. Moro, P8–13, P10–46, AvSYr10NIL, and the Avocet S are highly susceptible (ITs = 7–9). Wild-type Fielder and CB037 show moderate response (ITs = 4–6), characterized by obvious hypersensitive responses; however,YrNAMtransgenic Fielder#3 and CB037#5 are highly resistant (ITs = 1–2) lacking sporulation. This experiment was performed once for CYR33 and three times for CYR34 independently, with similar results. Stripe rust-susceptible Fielder and CB037 were transformed with YrNAM . Nine T 1 plants are shown on the left. P10–46 is the Pst -resistant control. Plants were inoculated with Pst race CYR32. c The integration (genomic DNA, or gDNA) and expression (cDNA) of YrNAM . Samples pair with those in ( b ). The target band for gDNA genotyping with primer pair YrNAM - F8R7 is 698 bp; the smaller band (572 bp) in P10–46 and CB037 is amplified from the chromosome 1D homolog, which does not have YrNAM . YrNAM - F4R43 was used for cDNA expression with a target band of 676 bp. The Pst test for T 1 plants using CYR32 was performed three times independently with similar results. Source data are provided as a Source Data file. Full size image Fig. 3: Reaction types of YrNAM -containing materials to the avirulent and virulent Pst races. a YrNAM -avirulent race CYR33. Moro, P8–13, P10–46, and AvSYr10NIL (AvS + Yr10 ), and YrNAM- transgenic Fielder#3 and CB037#5 are resistant with obvious HR (ITs = 2), while Avocet S (AvS) and the non-transformed Fielder and CB037 are susceptible (ITs = 7–9). b YrNAM -virulent race CYR34. Moro, P8–13, P10–46, AvSYr10NIL, and the Avocet S are highly susceptible (ITs = 7–9). Wild-type Fielder and CB037 show moderate response (ITs = 4–6), characterized by obvious hypersensitive responses; however, YrNAM transgenic Fielder#3 and CB037#5 are highly resistant (ITs = 1–2) lacking sporulation. This experiment was performed once for CYR33 and three times for CYR34 independently, with similar results. Full size image YrNAM is an ancient gene and is present in wild wheat species In Chinese Spring chromosome 1B (IWGSC, RefSeq v2.1), YrNAM is homologous to TraesCS1B03G0003600LC.1 and TraesCS1B03G0003500LC.1 , which are adjacent to the Yr10 diagnostic marker Xsdauw79 ( TraesCS1B03G0003800 ) [10] and around 1.0 Mb from TraesCS1B03G0000200 ( AF149112- corresponding gene) (Supplementary Fig. 3 ). The YrNAM homologs in chromosomes 1A and 1D were undetectable in RNA-Seq data from resistant WT P10–46, Moro, and the seven YrNAM -defective mutants. These homologs were only associated with low expression in public datasets (Supplementary Fig. 4 ). The phylogenetic analysis (Supplementary Figs. 5 and 6 , Supplementary Data 6 ) and molecular marker investigation (Supplementary Fig. 7 , Supplementary Data 7 ) revealed close homologs of YrNAM in Aegilops longissima and Ae. sharonensis , suggesting that the origin of YrNAM predates the speciation of wheat B- and D-subgenome progenitors, probably 7.3 million years ago [19] . The ZnF-BED domains were highly conserved among these YrNAM homologs, especially among genes annotated in chromosomes 1A, 1B, and 1S (Supplementary Fig. 8 ). In contrast, there was 37–44% identity between the YrNAM and the ZnF-BED domains of the six characterized NLR-BED genes for disease resistance in the Poaceae (Supplementary Fig. 8 ). The phylogenetic tree analysis showed the ZnF-BED domain of YrNAM is distinct from the ZnF-BED domains of NLR proteins in Poaceae (Supplementary Fig. 9 , Supplementary Data 8 ). Thus, the ZnF-BED domain insertion in YrNAM is independent of the ones in NLRs Rph15 and Yr5/Yr7. YrNAM is absent in most wheat lines To determine the distribution of YrNAM in cultivated wheat, we screened 60 AF149112- containing lines that were acquired from 659 wheat accessions [9] , [10] . Four lines (Fengmai 2, Fufan 24, Xianshixinmai, and Xiangnong 3) were positive for YrNAM-F8R7 (located at the 3′-end of YrNAM ) but negative for YrNAM-F1R3 (5′-end of YrNAM ) and YrNAM-F02R2 (internal region of YrNAM ) (Supplementary Fig. 10 , Supplementary Data 9 ). We then screened another panel of wheat germplasm, including 578 Chinese cultivars and advanced breeding lines and 59 Hungarian cultivars; YrNAM was not identified in any of them (Supplementary Data 10 ). The general absence of YrNAM in most wheat might be caused by its close linkage to an undesired trait, the brown glume locus Rg1 [20] . In this study, we used STAM, a simple and straightforward method for gene cloning in hexaploid wheat. It could be used in other plant species with complex genomes. STAM does not require a reference genome assembly; it only requires an Iso-Seq dataset from the WT and RNA-Seq data from multiple independent loss-of-function mutants that have a mutation in an exon. Our WT (F 7 generation) was homozygous, but in theory, STAM could be adapted for heterozygous plants. In addition, while we screened for EMS-type of mutations, the method could be useful for mutations such as small insertions or deletions generated by other mutagens. YrNAM is absent in most wheat cultivars, depriving the use of public genome assemblies to clone this gene as most of them are based on wheat cultivars. Alternatively, we can perform whole genome/chromosome sequencing of a WT with YrNAM to clone the gene. However, the cost of assembling a polyploidy genome like wheat is still high. Since STAM does not require whole genome/chromosome sequencing, it is a low-cost option for gene cloning. In addition, independent EMS mutants, which are required by STAM, are relatively easy to obtain in wheat, particularly when the trait is encoded by a single gene. Further, it is worth noting that the expression of YrNAM is low; we only detected 8 circular consensus sequencing (CCS) reads of YrNAM in 20 Gb Iso-Seq (~3.3 million CCS reads) from the WT, which translates to average 1.56–4.21 transcripts per million (TPM) in RNA-Seq of the WT at different time points after Pst inoculation. Thus, the success of cloning YrNAM indicates that STAM is feasible for cloning genes with low expression levels. However, STAM may not be a good option for cloning genes for polygenic traits. In addition, it is unsuitable for cloning genes with mutations in regulatory parts of a gene. Recently, a method called MutIsoSeq, which is similar to STAM, was developed to clone wheat leaf rust resistance gene Lr9 / Lr58 [21] . In comparison to MutIsoSeq, which keeps multiple Iso-Seq isoforms derived from the same gene, STAM employs a non-redundant full-length transcriptome as a reference. In addition, the MutIsoSeq protocol aims to sequence about 70 Gb RNA-Seq data for each Lr9 / Lr58 mutant [21] ; our study shows a smaller dataset of 15–18 Gb is sufficient for STAM. The success of cloning Lr9 / Lr58 and YrNAM indicates the effectiveness of using full-length transcripts instead of high-quality genome assembly as the reference for gene cloning. STAM and MutIsoSeq add to the toolbox for gene cloning in wheat and other species with complex genomes. These methods are effective when target genes are either located in recombination-suppressed regions, absent in the reference genome, or encoding non-NLRs. Till now, the Yr10 region harbors two genes responsible for stripe rust resistance, Yr10 CG and YrNAM , which are separated by around 1.0 Mb based on the Chinese Spring reference genome (Supplementary Fig. 3 ). Since there is no reference-quality genome assembly of Moro or P10–46 available, the exact distance and sequence between Yr10 CG and YrNAM in these two accessions are unknown. In the functional validation of Yr10 CG [8] , Moro plants that transfected with barley stripe mosaic virus (BSMV) constructs were susceptible to Pst race SRC-84; one transgenic line expressing Yr10 CG was resistant to SRC-84 but not to race CDL-29, which was detected in North America from 1983 to 1987 and was virulent on Moro [3] . Because Pst race CDL-29 was unavailable, we used Chinese yellow rust races (CYR), including CYR 29, CYR32, and CYR33, which are avirulent on Moro and WT P10–46, and CYR34, which is virulent on Moro and P10–46, for disease resistance assays. Transgenic Fielder and CB037 expressing YrNAM driven by its endogenous promoter are resistant to CYR 29, CYR32, CYR33, and CYR34. Without disease resistance assay using the historic North American strains such as CDL-29 that were used to characterize Yr10 , we cannot determine whether YrNAM is the original Yr10 or not. Regardless, the Wheat Gene Atlas [2] has called Yr10 CG a synonym for Yr10 . To avoid confusion, we name the gene conferring resistance to Pst strains CYR29, CYR32, and CYR33 as YrNAM . We also note that YrNAM may hold some of the breeding value that was previously attributed to Yr10 as it was considered the sole resistance in the region [22] . The dominant stripe rust resistance gene YrNAM encodes for two domains: 5′ NAM and 3′ ZnF-BED. Our mutational analysis suggests that both domains are required for stripe rust resistance. In alignments of YrNAM to available homolog sequences in public databases, the ZnF-BED domain is highly conserved (Supplementary Figs. 6 and 8 ), but the NAM domain is more divergent. Previously, the ZnF-BED domain was identified in several resistance genes to wheat stripe rust ( Yr5 and Yr7 ) [11] , barley leaf rust ( Rph15 ) [23] , and the rice bacterial pathogen Xanthomonas oryzae pv. oryzae ( Xa1 ) [24] and X. oryzae pv. oryzicola ( Xo1 ) [25] . However, besides the ZnF-BED domain, these resistance genes contain an NLR domain, which is absent in YrNAM . While the ZnF-BED domain in NLR might act as a decoy for pathogen effector [11] , [26] , the function of the ZnF-BED domain in the non-NLR YrNAM needs to be determined. Finally, we showed that YrNAM likely evolved before the speciation of wheat B- and D-subgenome progenitors. Since it is only present in a few wheat cultivars, there is potential for incorporating it into a wide variety of contemporary wheat cultivars for stripe rust-resistance breeding. Plant materials Yr10 single-gene lines, P8–13 and P10–46, were derived from an F 3 population of a cross between Pst -resistant cultivar Moro and Pst -susceptible cultivar ‘Huixianhong’ (HXH) [10] . P8–13 and P10–46 are homozygous in the Yr10 locus. The Yr10 mapping population, containing 126 F 2:3 siblings of P8–13 and P10–46 [10] , was used for linkage analysis of YrNAM in this study. In a fine mapping effort working with 7177 F 2:5 plants, 62 homozygous and susceptible recombinants were obtained in the Xpsp3000 - Xsdauw79 interval [10] . Thirty-seven of the recombinants were also tested by PCR for YrNAM . To determine the distribution of YrNAM , we tested a large collection of wheat germplasm: 60 Yr10 CG lines [9] , [10] (i.e., with Genbank accession AF149112, which, as shown here is approximately 1.0 Mb from YrNAM ); 578 Chinese wheat cultivars (advanced lines); 59 Hungarian cultivars released between 1970–2013; and 56 Ae. longissima and Ae. sharonensis accessions from the U.S. National Plant Germplasm System. Pst races A mixture of Pst spores that originally contained CYR29, CYR31, and CYR32 have been amplified in Taian, Shandong Agricultural University, and was used for field trials with the EMS mutants and growth chamber trials with the transgenic plants. The transgenic plants were additionally tested with the single race CYR32 and CYR33 provided by the Institute of Plant Protection, Chinese Academy of Agricultural Sciences, and CYR34 provided by the College of Plant Protection, Northwest A&F University, and a mixture of spores from naturally infected wheat fields in Luohe, Henan province, China (collected by Luohe Academy of Agricultural Sciences). EMS mutagenesis In 2016, about 10,000 seeds of P8–13 and P10–46, which were homozygous in Yr10 , were treated with EMS (Sigma-Aldrich Co., St. Louis, MO, USA). Both 1% (97 mM in water) and 1.05% (102 mM in water) were used to treat 5000 seeds. Each batch of 400 seeds (M 0 ) was soaked in 200 mL EMS solution in a 1-l flask, incubated on a shaker at 150 rpm at 25 °C for 10 h, and washed with running water at room temperature for 4 h; this protocol has a kill rate of approx. 75%. The processed seeds (M 1 ) were spread out on wet paper towels inside covered plastic boxes and germinated in a growth chamber at 25 °C and 16 h light. After one week, seedlings were transplanted into a greenhouse. A total of 2100 M 1 plants were harvested in June 2017. Every 10 M 1 plants were harvested as a pool, generating 211 pools (M1–M211). To identify Pst -susceptible mutants, 100 random M 2 seeds per pool were sowed in the field in Oct. 2017. In total, 14 segregating pools and 20 Pst -susceptible mutants were acquired. After confirming the Yr10 region by Xsdauw79 (a Yr10 co-segregating marker) [10] , we chose 12 Pst -susceptible mutants for further studies, including M16, M19, M38, M42, M52, M54, M62, M110, M160-1, M160-2, M168, and M175. Sequencing trait-associated mutations (STAM) For Iso-Seq of resistant WT P10–46, leaf tissues were sampled at 0 and 24 h after Pst infection. Total RNA was extracted using TRIzol reagent (Tiangen Biotech Co., Beijing, China) following the manufacturer’s protocol. RNA integrity was evaluated by Agilent 2100 Bioanalyzer (Agilent Technologies, CA, USA). Two micrograms of total RNA were used for first-strand cDNA synthesis and PCR amplification. Two sequencing libraries (0 and 24 h after Pst infection) were prepared using the Clontech SMARTer PCR cDNA Synthesis Kit (Clontech, Dalian, China) and then sequenced using the PacBio Sequel II system (PacBio, CA, USA). For whole-genome DNA resequencing of P10–46, DNA was isolated from uninoculated leaves using the standard CTAB method [27] . Genomic fragments (~250 bp) were prepared for Illumina NovaSeq (2 × 150 bp reads) and produced ~153 Gb raw data. Clean data were mapped to the Poaceae repeat element database mipsREdat 9.3p (PGSB Repeat Database) using BWA (version 0.7.17); unmapped reads (44.2 Gb, ~29%) were recovered using a homemade Perl script, and a de novo assembly was performed using SPADES v3.15 ( https://github.com/ablab/spades ). Wheat cultivar Moro and seven Pst -susceptible mutants (M16, M19, M38, M62, M110, M160-1, and M168) were sampled for RNA-Seq. Total RNAs were extracted using TRIzol reagent from leaf tissues 24 h post Pst inoculation. Standard indexed libraries were prepared and pooled for Illumina sequencing, producing ~18 Gb paired-end data per library. Iso-Seq, DNA resequencing, and RNA-Seq were performed by Berry Genomics (Beijing, China). The major steps of STAM are as below: (1) De novo transcriptome reconstruction. The raw sequencing reads (PacBio subreads) were processed by ccs to generate polished circular consensus sequence (CCS reads). After primer removal and demultiplexing using lima (version 2.2.0), IsoSeq3 ( https://github.com/PacificBiosciences/IsoSeq ) was used to trim PolyA tails and generate full-length, non-concatemer reads (FLNC reads); two SMRT cells FLNC reads were merged and clustered to generate polished transcript isoforms (HQ transcripts). (2) Construction of final transcriptome reference. HQ transcripts were mapped to the genome reference of Pst isolate 134E [28] using Minimap2 ( https://github.com/lh3/minimap2 ) to identify Pst contamination. After removing Pst transcripts, transposable elements were masked using RepeatMasker ( http://www.repeatmasker.org ) based on the repeat library Dfam3.6 ( https://www.dfam.org ). Afterward, clean HQ transcripts were mapped to wheat Chinese Spring genome reference IWGSC RefSeq v2.1 [29] using Minimap2 in order to produce aligned HQ transcripts. To collapse redundant isoforms caused by 5′ RNA degradation, Cupcake and Cogent ( https://github.com/Magdoll ) were used to generate unique transcripts for well-mapped reads and unmapped reads, respectively. Then, the two non-redundant transcript data were combined as a final transcript set using CD-HIT-EST with the sequence identity threshold at 100% (-c 1), resulting in 40,564 non-redundant transcripts that were used as references for variant calling. (3) Variant calling and rapid identification of a gene that confers a trait of interest. For RNA-Seq reads of Moro and Pst -susceptible mutants, adapter trimming, and quality filtration were performed using fastp ( https://github.com/OpenGene/fastp ); clean data was then mapped to transcript references from the previous step using STAR ( https://github.com/alexdobin/STAR ). Potential PCR-duplicated reads were also removed using Picard ( https://broadinstitute.github.io/picard ). SNPs were identified by the HaplotypeCaller tool of GATK v4.2 in GVCF mode ( https://gatk.broadinstitute.org ). Then, all the per-sample GVCFs were gathered and passed to GATK GenotypeGVCFs for joint calling. Variants were preliminarily filtered using GATK VariantFiltration with the parameter “DP < 5 | | FS > 60.0 | | MQ < 40.0 | | QD < 2.0”, which generated analysis-ready SNPs. Qualified SNPs met all the following conditions: (a) read depth ≥ 5; (b) homozygous site; (c) either a G → A or a C → T mutation; (d) the count of SNPs per transcript in each mutant = 1; and (e) scoreable in >60% (four of seven) of the mutants. Amongst all seven mutant lines, a total of 6516 reference transcripts were identified with one or more G → A and/or C → T mutations. Genetic transformation of wheat To construct a vector to express YrNAM with its endogenous promoter, we amplified a 5358 bp genomic fragment, which contains 2577 bp before ‘ATG’ to 616 bp after ‘TAA’ in contig NODE_33935, using DNA from P10–46, high-fidelity polymerase Phanta Max (Vazyme Biotech, Nanjing, China) and PCR primers F09 and OL-R3. The resultant fragment was cloned into the pENTR vector using a pBM27 toposmart cloning kit (Biomed, Beijing, China). Using LR Clonase™ II (Invitrogen, Waltham, USA), the YrNAM native gene was then cloned into PC613, which has 35S:: Bar for plant selection. The final construct PC1213 was transformed into Agrobacterium strain EHA105. Genetic transformation of common wheat was carried out by Agrobacterium -mediated transfer [30] . Two wheat genotypes susceptible to stripe rust, Fielder and CB037, were used as recipients. Plants were grown in a growth chamber with 16 h light at 24 °C and 8 h darkness at 18 °C. T 0 transgenic plants were genotyped by amplifying Bar (Bar-F/R) and YrNAM (F8/R7). Pst inoculation Moro, P10-46, HXH, Fielder, CB037, and EMS mutants (M 2, M 3 ), transgenic plants (T 1 and T 2 ), and selected recombinants (F 2:5 ) were tested for seedling resistance to Pst races. M 2 EMS mutants were tested in the field with a mixture of spores of CYR29, CYR31, and CYR32. In total, 211 pools (10 M 2 lines per pool) were planted as pool-based rows in fall 2017 and were inoculated in spring 2018 at tillering stage (Zadoks stage 31) [31] . To inoculate, a 2.5 mL syringe was used to inject an aqueous spore suspension into the leaf bundles, totaling three sequential injections at 7 d intervals. To maintain moisture, mild irrigation followed each inoculation. Susceptible mutants were screened 4–6 wk post inoculation when the control plants of HXH showed full susceptibility to Pst . Pst tests for other materials were carried out in growth chambers. Inoculations were performed at the seedling stage (Zadoks stage 11–13) [31] by injecting spore suspension into the leaf bundles or by applying a mixture of spores and talc (or Lycopodium ) powder onto the leaf surface. Inoculated seedlings were kept at 10 °C and 100% relative humidity and in darkness for 24 h, and were then shifted to 16 h light at 15 °C and 8 h darkness at 10 °C. Infection types (ITs) were recorded 15 days post inoculation using a 0–9 scale, where ITs 0–3 were considered resistant, 4–6 intermediate, and 7–9 susceptible [3] . Phylogenetic analysis Homologs of YrNAM in common wheat and related species were acquired by blasting the YrNAM transcripts against the current Triticeae genomes in WheatOmics ( http://wheatomics.sdau.edu.cn/ ). Multiple sequence alignments were performed using MAFFT v7.475 L-INS-I ( https://mafft.cbrc.jp/alignment/software/ ) with default parameters. Poorly aligned sequences were removed before constructing a tree. A phylogenetic tree was built by the approximately maximum-likelihood method using FastTree ( http://www.microbesonline.org/fasttree/ ) with default parameters. Cellular localization A GFP fusion construct (PC1221, Ubi:: GFP : YrNAM ) was prepared by amplifying the YrNAM CDS from P10-46 with the YrNAM -F13/R13 PCR primers and the GFP CDS from pMDC43 [32] using the GFP-F12/R12 primers. The primers GFP-F12, -R12, and YrNAM -R13 each contained a 17-20 bp fragment for homologous recombination. The GFP and YrNAM were fused and ligated to BsrG I linearized PC186 [33] using ClonExpress® MultiS One Step Cloning Kit (C113, Vazyme, Nanjing, China). The resultant PC1221 was then transformed into Agrobacterium strain EHA105. PC1221 in EHA105 was transiently expressed in tobacco ( Nicotiana benthamiana ) leaves using the infiltration method. After 48 h growth in a controlled environment with a long day photoperiod, the tobacco leaves were photographed using a confocal microscope (Zeiss LSM 880 NLO, Germany). Three views were captured for each target cell, including a bright field, a GFP channel, and a channel for 4′,6-diamidino-2-phenylindole dihydrochloride (DAPI). GFP expression vector pzp211-GFP was used as a control. Reporting summary Further information on research design is available in the Nature Portfolio Reporting Summary linked to this article.